Transcription factor binding kinetics constrain noise suppression via negative feedback Negative autoregulation, where a transcription factor regulates its own expression by preventing transcription, is commonly used to suppress fluctuations in gene expression. Recent single molecule in vivo imaging has shown that it takes significant time for a transcription factor molecule to bind its chromosomal binding site. Given the slow association kinetics, transcription factor mediated feedback cannot at the same time be fast and strong. Here we show that with a limited association rate follows an optimal transcription factor binding strength where noise is maximally suppressed. At the optimal binding strength the binding site is free a fixed fraction of the time independent of the transcription factor concentration. One consequence is that high-copy number transcription factors should bind weakly to their operators, which is observed for transcription factors in Escherichia coli . The results demonstrate that a binding site’s strength may be uncorrelated to its functional importance. The number of molecules in a biological cell is always fluctuating because of the probabilistic nature of chemical reactions [1] , [2] . Negative feedback is therefore commonly used to maintain homeostasis and to reduce the fluctuations in intracellular processes such as gene expression [3] , [4] , [5] . For example, nearly half of the ~300 transcription factors (TFs) in Escherichia coli make use of negative feedback on their own expression [6] , [7] . However, the chemical noise that makes regulation necessary also limits the accuracy of feedback regulation [8] . For this reason, we need to consider the physical limitations in how feedback systems can be implemented by chemical components when analysing optimal strategies for suppressing noise in gene expression [9] . Recent single molecule in vivo measurements show that it takes much longer time for a TF molecule to find its chromosomal operator site than what is expected from in vitro measurements. The discrepancy is due to slow intracellular diffusion, significant binding to non-specific DNA and that chromosomal DNA is crowded by other proteins [10] . As a consequence, it takes about 4 min for a single LacI repressor molecule to find and bind a single lac operator in the E. coli chromosome [11] . The slow association kinetics, as quantified by a low association rate constant k a , implies that the dissociation rate from the operator has to be low (low k d ) to accomplish strong feedback with a high binding constant K = k a / k d . However, k d also sets the time scale for how often the feedback system samples the cellular concentration that should be regulated. We should therefore ask if transcriptional noise is better suppressed with fast or strong negative feedback. Modelling slow TF binding The consequences of limited TF-binding rates can be modelled by the basic steps in expressing a TF gene and the TF binding to the DNA [12] , [13] , [14] , [15] , [16] , [17] , [18] , [19] , illustrated in Fig. 1 . In summary, an active gene is transcribed into mRNA, the mRNA is translated into a repressor protein several times or degraded, and the repressor binds the operator site mediating the negative feedback or is degraded. When the operator is bound the gene is inactive until the repressor dissociates. We now ask what dissociation rate leads to optimal noise suppression when the average expression level is maintained constant by compensating stronger repression with higher transcription rate. By posing the optimization problem in this way, we implicitly assume that the purpose of the negative feedback system is to maintain a certain concentration of the regulated protein, and that the parameters that evolution can work with are the strength of the promoter and the strength of repressor binding. 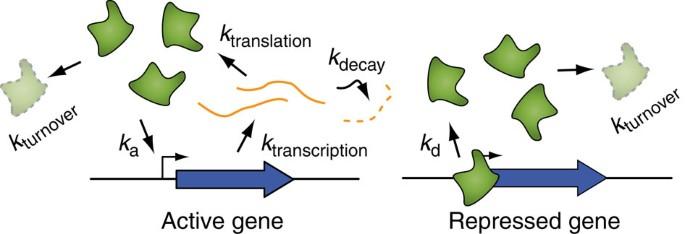Figure 1: The negative feedback motif. The TF protein binds the regulatory region of its own gene and suppresses expression at high TF concentration. The rate constant for bindingkais limited by the complex process of finding a specific site in the genome, whereas the dissociation ratekdcan be very high at the expense of poor binding strength. At lowkd, the TF binds strongly and the mean response in the regulation is sensitive. However, when considering the discrete nature of chemical reaction, a lowkdimplies that the TF dissociates rarely and that all mRNAs are made in bursts at these events. Figure 1: The negative feedback motif. The TF protein binds the regulatory region of its own gene and suppresses expression at high TF concentration. The rate constant for binding k a is limited by the complex process of finding a specific site in the genome, whereas the dissociation rate k d can be very high at the expense of poor binding strength. At low k d , the TF binds strongly and the mean response in the regulation is sensitive. However, when considering the discrete nature of chemical reaction, a low k d implies that the TF dissociates rarely and that all mRNAs are made in bursts at these events. Full size image It is straightforward to perform stochastic simulations corresponding to the reaction system in Fig. 1 (ref. 20 ). The results of such simulations are displayed in Supplementary Fig. S1 and will serve as reference point for the mathematical analysis. The fluctuations are quantified using the variance, σ 2 , to mean, <x>, ratio VMR=σ 2 /<x>. As we fix the average number of molecules <x> for varying feedback, finding an optimal k d in terms of minimizing the VMR is thus equivalent to optimize noise in terms of the coefficient of variation σ 2 /<x> 2 or the s.d. over the mean σ/<x>. In Fig. 2a , we show that the VMR has a minimum with respect to the dissociation rate k d . Higher dissociation rates imply weak binding, insensitive regulation and small noise suppression. Lower dissociation rates imply that mRNAs have to be made in noisy bursts to maintain the average protein expression level despite rare dissociation events. This inevitable property of negative transcriptional autoregulation is lost in the quasi steady state (QSS) assumption where it is assumed that the TF binding equilibrates rapidly in its binding to operator sites. The QSS assumption leads to the misconception that stronger binding, compensated by a strong promoter to maintain constant copy number, results in more sensitive regulation and better noise suppression. The reason for the error is that the slow TF kinetics that follows with strong feedback is in conflict with the QSS assumption. In Supplementary Fig. S2 , the discrepancy for strong feedback is shown, an effect that is previously demonstrated in comparisons with simulations [16] . 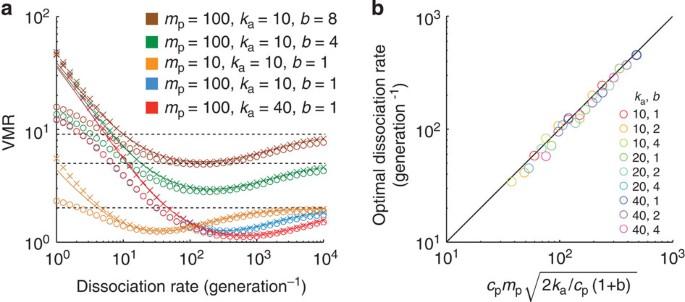Figure 2: Optimal dissociation rate of negative autoregulation. The left panel (a) displays the VMR as a function of the dissociation rates (kd), for various average amount (mp) of the regulated TF protein, TF association rate per operator (ka) and average numbers of TFs made per mRNA (b=ktranslation/kdecay). The solid lines are the analytical expressions given in theSupplementary Note 1. The crosses are measurements from stochastic simulations of fixed size cells where cell growth is approximated with protein decay. Circles are measurements from stochastic simulations of cells that are growing, replicating and dividing with measurements taken in the middle of the cell cycle. Rates are defined in terms of the generation time and TFs are only diluted by cell growth. In addition to the parameters given in the figure, the mRNA lifetime is 1/10 of the generation time. The dashed lines are VMR of unregulated synthesis. In the right panel (b), we display how the expression in Equation 3 for the optimal dissociation rate compares with that obtained from simulations of exponentially growing cells for specific parameter combinations (inset), each with three different mean protein copy numbers (20, 40 and 80). Note that the VMR is approximated in the middle of the cell cycle (seeSupplementary Note 1). Figure 2: Optimal dissociation rate of negative autoregulation. The left panel ( a ) displays the VMR as a function of the dissociation rates ( k d ), for various average amount ( m p ) of the regulated TF protein, TF association rate per operator ( k a ) and average numbers of TFs made per mRNA ( b=k translation / k decay ). The solid lines are the analytical expressions given in the Supplementary Note 1 . The crosses are measurements from stochastic simulations of fixed size cells where cell growth is approximated with protein decay. Circles are measurements from stochastic simulations of cells that are growing, replicating and dividing with measurements taken in the middle of the cell cycle. Rates are defined in terms of the generation time and TFs are only diluted by cell growth. In addition to the parameters given in the figure, the mRNA lifetime is 1/10 of the generation time. The dashed lines are VMR of unregulated synthesis. In the right panel ( b ), we display how the expression in Equation 3 for the optimal dissociation rate compares with that obtained from simulations of exponentially growing cells for specific parameter combinations (inset), each with three different mean protein copy numbers (20, 40 and 80). Note that the VMR is approximated in the middle of the cell cycle (see Supplementary Note 1 ). Full size image Optimal binding strength To understand how the noise relates to the binding strength, we need to solve the chemical master equation [21] for the well-stirred system corresponding to the reaction network in Fig. 1 . The molecules are considered to be well-mixed in the cell since the search time of finding the binding site is of the order of minutes and proteins diffuse across the cell on the order of seconds. Possible effects of diffusion noise are neglected [22] . We derive an expression for the variance in the number of repressor molecules, see Methods section and Supplementary Note 1 , where a key step is to approximate third order moments in terms of lower order moments. In Fig. 2a we display the analytical solution for the VMR, solid lines and simulation results for the complete system. As a reference, we display the VMR of unregulated protein synthesis (dashed line), which is approached in the limit of no feedback and given by [13] , [14] where b is the average number of proteins made per mRNA molecule. Noise is suppressed below the unregulated level, VMR 0 , when the dissociation rate is higher than k d,min . where c p is the rate of protein turnover, which can be a combination of dilution and degradation, m p is the mean number of repressor protein molecules and c p m p is therefore equal to the average rate of protein synthesis. See Supplementary Note 2 for details. When several proteins are made per mRNA ( b »1), Equation 2 implies that the repressor has to dissociate at a rate corresponding to the protein synthesis rate divided by the number of proteins made per mRNA. This result makes sense, as the mRNAs otherwise would have to be made in bursts. The denominator is 1+ b , and not b , as it is sufficient that the repressor dissociates at the rate of protein synthesis, c p m p , to maintain the uncorrelated protein synthesis events, even if b <1. High-copy number E. coli TF exists in numbers up to several thousands [23] , [24] , [25] . If we consider as an example a high-copy number TF to be made at a rate of 1,000 molecules per generation and with b=8 , the median for E. coli [26] , the TF needs to dissociate more than 100 times per generation or negative feedback adds more noise than the unregulated situation. In order to gain noise suppression by the regulation, the transcription events should not only be uniformly distributed in time, which is the case for unregulated synthesis, but respond to deviations from the average value. For this reason, the operator binding state has to be given some time to equilibrate to free protein concentration between expression events. We find that the optimal dissociation rate is where k a is the association rate for the repressor to a single operator site. See Supplementary Note 2 for details. In Fig. 2b , we show that equation 3 describes the optimal dissociation rate for all relevant parameters by comparing the equation with the optimal dissociation rate obtained from fully stochastic simulations of growing cells. The result can also be described in terms of the fraction of time the operator should be free, that is, where the search time of the TF, τ s =1/ k a , and the protein turnover time, τ G =1/ c p . For example, if the search time is 4 min, which is close to the physical limit [11] , the generation time is 22 min and b =8, the operator should be free 17% of the time independent of the number of regulated protein molecules. A highly abundant autorepressor TF should therefore bind weakly to its operator. With the previous example of 1,000 molecules, Equation 3 gives that a TF should (roughly) be bound on average one second before dissociating for optimal noise suppression. Global TF-binding sequence statistics In E. coli , the expression of 51% of all genes are under control of seven highly expressed global transcriptional regulators (CRP, FNR, IHF, FIS, ArcA, NarL and Lrp). Among these all but ArcA are employing negative feedback on their own synthesis [6] , [7] . However, all the six TFs bind weakly to the operators mediating the feedback compared with their binding to other specific sites ( Fig. 3 ), where the binding strengths are estimated using the heterology index [27] , [28] . The heterology index is for a given TF-binding site an estimation of the total reduction of binding free energy compared with if each base pair would be occupied by the most representative base pair in a set of recognition sites for the TF. The observed weak autorepressor binding sites cannot be explained from the need of having a high expression of the TFs, as the same expression level could be achieved by a combination of stronger promoters and stronger feedback. Instead, the results from our calculations demonstrate another explanation; the binding sites need to be weak to keep them free a significant fraction of the time despite the high concentration of these TFs. 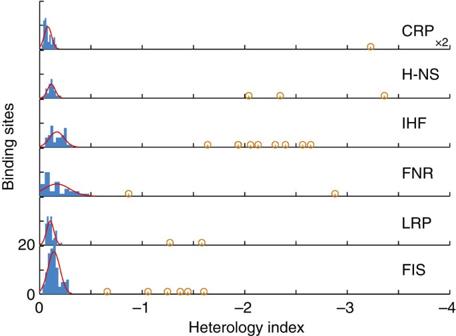Figure 3: Global regulators show weak autorepressor binding. The figure displays the histograms of the binding site heterology index for six of the seven global regulators controlling 51% of the genes inE. coli. The blue bars display the histogram of the heterology index of the forward repressor binding sites, that is, sites in the promoter of other genes. The orange markers correspond to the heterology index of the repressor binding sites in the promoter of the regulators’ own gene. The absolute heterology index is proportional to the reduction in binding energy compared with consensus binding sequence. The red lines are fitted normal distributions of the histograms of the forward repressor bindings. Figure 3: Global regulators show weak autorepressor binding. The figure displays the histograms of the binding site heterology index for six of the seven global regulators controlling 51% of the genes in E. coli . The blue bars display the histogram of the heterology index of the forward repressor binding sites, that is, sites in the promoter of other genes. The orange markers correspond to the heterology index of the repressor binding sites in the promoter of the regulators’ own gene. The absolute heterology index is proportional to the reduction in binding energy compared with consensus binding sequence. The red lines are fitted normal distributions of the histograms of the forward repressor bindings. Full size image Recently Lestas et al . [8] derived a fundamental limit for noise suppression in a feedback control system. When applied to the case where the regulated quantity itself is mediating the feedback, there is no information loss between making the species and regulating its production and the noise can therefore theoretically be suppressed to zero. Such feedback would be implemented by having infinite synthesis rate when the copy number is below the set point and zero synthesis when the copy number is at the set point or higher. However, in practice the physical implementation of the control systems implies that gene expression cannot be controlled this accurately. For example, although the repressor is bound to the operator, the copy number can fall below the set point without the control system being able to respond. In order to determine and respond to the copy number deviations, the TF has to dissociate such that the rebinding time can be used as a measure of the free concentration. The rebinding time will, however, be exponentially distributed and information is lost by making a decision based on a single-rebinding event. To estimate the concentration accurately in the system, the repressor has to bind and dissociate several times for each synthesis event such that the average occupancy at the time scale of the gene expression accurately reflects the concentration in the cells. Related constraints for optimal information transmission in gene regulatory systems where a signal molecule is regulated by upstream regulators have previously been analysed [29] and how feedback may improve the fidelity in transmission of time-varying signals [30] . In summary, we have derived the optimal dissociation rate for the case of a single auto-regulatory repressor protein and in the Supplementary Fig. S2 we demonstrate that the same principles apply for cooperative repression schemes. Based on these results, we conclude that there is no reason to consider weak-binding sites as unimportant. On the contrary, for regulatory fidelity by abundant TFs it is critical that binding is weak. Solving the moment equations The first and second moments at stationary conditions have been calculated from the chemical master equation by performing two moment closure steps, where third order moments are approximated with lower order moments (see Supplementary Note 1 ). After the approximation steps are performed, the second moment M pp of the protein copy number is shown to satisfy the cubic equation where and The cubic equation can be solved using Cardano’s method and the second moment M pp will depend upon the mean protein number m p , the protein turnover rate c p , the number of proteins translated per mRNA b , the binding association rate k a and the dissociation rate k d . The VMR of the protein copy number can be calculated from the second moment as Finding the optimal dissociation rate The dissociation rate k d,opt that minimize the VMR can be obtained by differentiating the cubic equation (5) with respect to k d and setting the derivative of M pp to zero (see Supplementary Note 2 ). How to cite this article: Grönlund, A. et al . Transcription factor binding kinetics constrain noise suppression via negative feedback. Nat. Commun . 4:1864 doi: 10.1038/ncomms2867 (2013).